Structural insights into 5′ flap DNA unwinding and incision by the human FAN1 dimer Human FANCD2-associated nuclease 1 (FAN1) is a DNA structure-specific nuclease involved in the processing of DNA interstrand crosslinks (ICLs). FAN1 maintains genomic stability and prevents tissue decline in multiple organs, yet it confers ICL-induced anti-cancer drug resistance in several cancer subtypes. Here we report three crystal structures of human FAN1 in complex with a 5′ flap DNA substrate, showing that two FAN1 molecules form a head-to-tail dimer to locate the lesion, orient the DNA and unwind a 5′ flap for subsequent incision. Biochemical experiments further validate our model for FAN1 action, as structure-informed mutations that disrupt protein dimerization, substrate orientation or flap unwinding impair the structure-specific nuclease activity. Our work elucidates essential aspects of FAN1-DNA lesion recognition and a unique mechanism of incision. These structural insights shed light on the cellular mechanisms underlying organ degeneration protection and cancer drug resistance mediated by FAN1. FAN1 possesses 5′ flap endonuclease and 5′-3′ exonuclease activities and is involved in a DNA ICL damage repair pathway [1] , [2] , [3] , [4] , [5] , [6] . FAN1 is thought to be recruited to ICLs via its interaction with the monoubiquitinated form of the FANCI-FANCD2 complex, and, accordingly, disruption of the nuclease activity of FAN1 sensitizes cells to ICL inducing agents [1] , [2] , [3] , [4] , [5] , [6] . In ICL repair, FAN1 is thought to co-operate with other nucleases to introduce DNA incisions necessary for the efficient unhooking of the ICL [1] , [2] , [3] , [4] , [5] , [6] . Interestingly, FAN1 inactivation can lead to chronic kidney diseases [7] and autism/schizophrenia [8] , linking defective DNA lesion repair with ageing [9] and neurological disorders [8] . Besides its positive role in genome maintenance, FAN1 is also implicated in conferring chemo-resistance in several cancer subtypes [10] , [11] , presenting itself as a promising drug target against chemotherapy resistance. Although the structures of viral/bacterial homologues of the FAN1 nuclease domain, VRR_NUC, are available [12] , neither the DNA interaction mechanism nor the exact role of human FAN1 in the ICL repair reaction is clear. Here we report three crystal structures of human FAN1 bound to 5′ flap DNA and provide biochemical data to elucidate FAN1-DNA substrate interplay. We show that FAN1 forms an asymmetrical dimer to engage the DNA lesion, unwind the flap and incise the unwound DNA intermediate. These results illustrate a highly unusual mode of DNA substrate engagement by FAN1 and provide insights into the critical role of FAN1 in ICL repair and in the prevention of functional decline in different organs. Moreover, our results should facilitate efforts directed at counteracting FAN1-mediated chemotherapy resistance in cancer treatment. Overview of FAN1-DNA complex A stable fragment [5] of FAN1 containing residues 373 to 1,017 (FAN1 373-1,017 ) was used for structural studies, as it covers all the essential domains for DNA processing and preserves near wild-type nuclease activity [5] . For crystallization, a DNA substrate with a one-nucleotide (1-nt) 5′ flap flanked by two duplex regions of 10 bp, designated as 5′-flap (10-1-10), was mixed with FAN1 373-1,017 carrying an active-site mutation [2] D960A to prevent DNA cleavage. 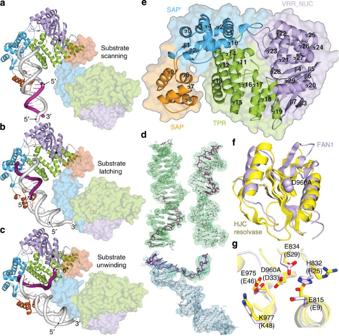Figure 1: The crystal structures of the FAN1-DNA complex. (a) The ‘substrate-scanning’ form with the FAN1 domains coloured: SAP in orange, SAP′ in cyan, TPR in green and VRR-NUC in violet. The active site is marked by a black star. The two FAN1 molecules in the dimer are in ribbon and surface presentations, respectively. The DNA is shown as coils (the flap strand in magenta with the flap position marked by a black arrow). (b) The ‘substrate-latching’ and (c) the ‘substrate-unwinding’ forms in the same scheme as in (a). (d) The unbiased electron density (simulated annealing omit maps) for the DNA substrates. mFo-DFc maps (2.0σ contour level) are shown as green meshes and 2mFo-DFc map (0.8σ) as blue meshes. The DNA is shown as sticks. Top left: ‘substrate-scanning’ form; top right: ‘substrate-latching’ form; bottom panel: ‘substrate-unwinding’ form. (e) Ribbon representation of FAN1 under a semi-transparent surface with the secondary structure elements labelled. (f) The overall and (g) the close-up views of the overlay of HJC resolvase domain (yellow, PDB 1GEF) and the FAN1 nuclease domain (violet). The side chain of active-site mutation D960A is highlighted as spheres in (f). The active site residues are labelled (HJC sequence in parenthesises) in (g). The duplex regions contained 1-nt (A or T) overhangs to facilitate crystallization (sequences in Supplementary Table 1 ). Three different crystal forms of FAN1 373-1,017 in complex with the 5′ flap DNA were obtained and they diffracted to resolutions of 2.2 Å (space group P2 1 2 1 2 1 ), 3.8 Å (P3 1 ) and 4.2 Å (P3 1 ), respectively. The structures were solved by the single-wavelength anomalous diffraction (SAD) method using signals from iodide ions, which were included in the crystallization buffer for the P2 1 2 1 2 1 crystal form, and subsequently by the molecular replacement method for the P3 1 crystals ( Table 1 ). All three structures were refined to good statistics with excellent geometry ( Table 1 ). Unambiguous electron density in the three crystal forms clearly reveals three distinct DNA conformations in the cleft formed by two FAN1 molecules ( Fig. 1a–d and Supplementary Fig. 1 ). Table 1 Data collection and refinement statistics. Full size table Figure 1: The crystal structures of the FAN1-DNA complex. ( a ) The ‘substrate-scanning’ form with the FAN1 domains coloured: SAP in orange, SAP′ in cyan, TPR in green and VRR-NUC in violet. The active site is marked by a black star. The two FAN1 molecules in the dimer are in ribbon and surface presentations, respectively. The DNA is shown as coils (the flap strand in magenta with the flap position marked by a black arrow). ( b ) The ‘substrate-latching’ and ( c ) the ‘substrate-unwinding’ forms in the same scheme as in ( a ). ( d ) The unbiased electron density (simulated annealing omit maps) for the DNA substrates. mFo-DFc maps (2.0σ contour level) are shown as green meshes and 2mFo-DFc map (0.8σ) as blue meshes. The DNA is shown as sticks. Top left: ‘substrate-scanning’ form; top right: ‘substrate-latching’ form; bottom panel: ‘substrate-unwinding’ form. ( e ) Ribbon representation of FAN1 under a semi-transparent surface with the secondary structure elements labelled. ( f ) The overall and ( g ) the close-up views of the overlay of HJC resolvase domain (yellow, PDB 1GEF) and the FAN1 nuclease domain (violet). The side chain of active-site mutation D960A is highlighted as spheres in ( f ). The active site residues are labelled (HJC sequence in parenthesises) in ( g ). Full size image The FAN1 373-1,017 molecule has three domains ( Fig. 1e ): a SAP containing domain as the primary DNA-binding domain, a TPR domain mediating inter-domain interaction and part of the dimerization interface and a VRR_NUC domain that harbours the catalytic site. The SAP domain consists of a canonical SAP fold and a SAP′ region that connects to the TPR domain. The VRR_NUC domain has similar fold and active site residues as the Achaea Holliday Junction resolvase HJC [13] , with a Cα root-mean-square deviation (RMSD) of 2.2 Å ( Fig. 1f,g ). This indicates a similar mechanism of metal-mediated catalysis, even though no metal ion is present here due to the mutation of the metal-coordinating residue D960A. A comparison with the HJC structure suggests that the DNA substrate is oriented at the active site by residues K977/H832 (K48/R25 in HJC) for hydrolysis mediated by residues E815/E834/D960/E975 (E9/S29/D33/E46 in HJC) ( Fig. 1g ). Consistent with the published data [2] , [3] , [5] , [6] , [14] , [15] , wild-type FAN1 373-1,017 exhibits strong endonuclease activity on 5′ flap DNA substrates, generating two endonuclease products at the fourth nt into the duplex region 3′ to the branch site and at the seventh nt into the single-strand (ss) region 5′ to the branch site ( Supplementary Fig. 2 ). It also exhibits exonuclease activity on 5′ flap, 3′ flap and double-stranded (ds) DNA substrates ( Supplementary Fig. 2 ). DNA promoted dimerization of FAN1 Two FAN1 molecules act together to recognize the DNA substrate. FAN1 alone is monomeric in solution [12] ; however, DNA binding promotes FAN1 dimerization in solution ( Supplementary Figs 3d and 8 ). Consistently, our crystal structures reveal DNA-induced assembly of a ‘head to tail’ FAN1 dimer via the TPR and NUC domains of the first FAN1 molecule interacting with the SAP domain of a second FAN1 ( Fig. 1a–c ). FAN1 dimer–DNA interactions are observed in all three crystals, each with a distinct DNA-binding form ( Fig. 1a–c ). These include (i) a ‘substrate-scanning form’ (P2 1 2 1 2 1 crystal) wherein the DNA contacts one of the FAN1 molecules in the dimer ( Fig. 1a ), (ii) a ‘substrate-latching form’ (P3 1 crystal 1) wherein the DNA becomes engaged with both FAN1 molecules ( Fig. 1b ) and (iii) a substrate ‘unwinding-form’ (P3 1 crystal 2) where the DNA interacts extensively with both FAN1 molecules and the flap-containing strand is unwound and points towards the active site ( Figs 1c and 2a ). Within the asymmetric dimer, one FAN1 molecule (denoted as P FAN1) appears to play a primary role in catalysis by engaging the DNA in its active site and the other FAN1 molecule (denoted as A FAN1) plays an auxiliary role, facilitating substrate orientation and flap unwinding. P FAN1 and A FAN1 in all crystal forms are structurally similar, with the Cα RMSD of 0.8~1 Å. Interestingly, an asymmetric arrangement of two MRE11 molecules has been observed in the structure of the MRE11-DNA complex [16] that functions in DNA double-strand break repair and signalling pathways, suggesting a similar strategy is employed for both enzymes to engage the DNA substrate and to prepare it for endonucleolytic incision. 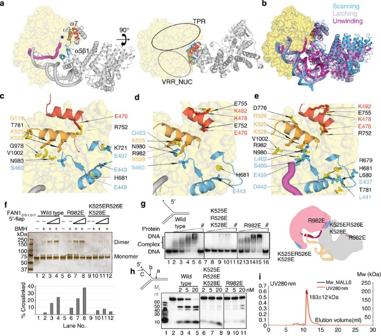Figure 2: The DNA-promoted dimerization of FAN1. (a) Orthogonal views of the ‘substrate-unwinding’ complex withPFAN1 as a yellow surface andAFAN1 as grey ribbons. The dimerization modules ofAFAN1 are highlighted with α7in light orange, α9in dark-orange and α5β1in cyan. The DNA is in grey with the flap-containing strand in magenta. The active site is marked by a black star. The TPR and VRR_NUC domains are marked by black ovals. (b) Superposition of the structures of the three FAN1-DNA forms. Main chains ofPFAN1 are aligned and shown as yellow surfaces, while the corresponding DNA andAFAN1 are in indicated colours. (c–e) Close-up views of detailed interactions at the dimer interface ((c) ‘substrate-scanning’ form, (d) ‘substrate-latching’ form and (e) ‘substrate-unwinding’ form). Residues involved are shown as sticks and labelled with the same colours as those of the secondary structures. (f) BMH crosslinking assay showing 5′-flap DNA-induced dimerization of FAN1373-1,017and its mutants as marked. Positions for FAN1373-1,017monomer and dimer are indicated. Top: silver-stained gel image; bottom: quantification of crosslinked protein as percentage of total protein input. (g) Bottom: DNA mobility shift assay of FAN1373-1,017and its dimerization mutants. Deproteinized DNA controls are labelled as #. Top inset: schematic summary of the locations of the mutations included in this figure. (h) Nuclease assay of FAN1373-1,017and its dimerization mutants using a 5′ flap DNA substrate, 2, 5, 20 nM of FAN1373-1,017and its dimerization mutants are used in the reaction. The endo- and exonuclease products are indicated as a, b and c shown in the schematic (top left). Quantifications of (g) and (h) are shown inSupplementary Fig. 3. (i) SEC-MALLS assay of FAN373-1,017D960A with DNA. FAN1373-1,017D960A and 5′flap DNA mixture (50 μM protein, 25 μM 5′flap (10-1-10) DNA, 100 μl) was resolved in a Superdex200 size exclusion column in buffer. Both UV absorption (red trace) and molecular weight (Mw) measurement (black trace) are shown (lefty-axis: UV absorption, righty-axis: calculated Mw,x-axis: elution volume). Figure 2: The DNA-promoted dimerization of FAN1. ( a ) Orthogonal views of the ‘substrate-unwinding’ complex with P FAN1 as a yellow surface and A FAN1 as grey ribbons. The dimerization modules of A FAN1 are highlighted with α 7 in light orange, α 9 in dark-orange and α 5 β 1 in cyan. The DNA is in grey with the flap-containing strand in magenta. The active site is marked by a black star. The TPR and VRR_NUC domains are marked by black ovals. ( b ) Superposition of the structures of the three FAN1-DNA forms. Main chains of P FAN1 are aligned and shown as yellow surfaces, while the corresponding DNA and A FAN1 are in indicated colours. ( c – e ) Close-up views of detailed interactions at the dimer interface (( c ) ‘substrate-scanning’ form, ( d ) ‘substrate-latching’ form and ( e ) ‘substrate-unwinding’ form). Residues involved are shown as sticks and labelled with the same colours as those of the secondary structures. ( f ) BMH crosslinking assay showing 5′-flap DNA-induced dimerization of FAN1 373-1,017 and its mutants as marked. Positions for FAN1 373-1,017 monomer and dimer are indicated. Top: silver-stained gel image; bottom: quantification of crosslinked protein as percentage of total protein input. ( g ) Bottom: DNA mobility shift assay of FAN1 373-1,017 and its dimerization mutants. Deproteinized DNA controls are labelled as #. Top inset: schematic summary of the locations of the mutations included in this figure. ( h ) Nuclease assay of FAN1 373-1,017 and its dimerization mutants using a 5′ flap DNA substrate, 2, 5, 20 nM of FAN1 373-1,017 and its dimerization mutants are used in the reaction. The endo- and exonuclease products are indicated as a, b and c shown in the schematic (top left). Quantifications of ( g ) and ( h ) are shown in Supplementary Fig. 3 . ( i ) SEC-MALLS assay of FAN 373-1,017 D960A with DNA. FAN1 373-1,017 D960A and 5′flap DNA mixture (50 μM protein, 25 μM 5′flap (10-1-10) DNA, 100 μl) was resolved in a Superdex200 size exclusion column in buffer. Both UV absorption (red trace) and molecular weight (Mw) measurement (black trace) are shown (left y -axis: UV absorption, right y -axis: calculated Mw, x -axis: elution volume). Full size image A conserved dimerization mode with some degree of variation is observed in the three FAN1-DNA structures, with the α 9 , α 7 and α 5 β 1 region of the A SAP domain lodging onto the surface in-between P VRR_NUC and P TPR ( Fig. 2a,b ). The helix α 9 seems to serve as a central core interaction module, while α 7 and α 5 β 1 adjust their positions and orientations to adapt to different dimer orientations ( Fig. 2c–e ). These interactions are mostly electrostatic in nature, including extensive hydrogen bonds and salt bridges between the two FAN1 molecules. Notably, a more extensive interface is seen in the ‘unwinding form’ wherein the two FAN1 molecules associate more tightly to unwind the 5′ flap DNA. We carried out mutagenesis to validate the observed dimer interface ( Fig. 2f–h and Supplementary Figs 2e and 3 ). As predicted from the dimer structure, a triple mutation K525E/R526E/K528E on the core α 9 interface greatly diminished DNA-induced dimerization as revealed by protein crosslinking using the chemical reagent BMH (bis(maleimido)hexane) ( Fig. 2f ), size-exclusion chromatography (SEC, Supplementary Fig. 3e ) and SEC-multi angle lase light scattering (SEC-MALLS, Fig. 2i ). As a consequence, the substrate-binding affinity to 5′ flap DNA ( Fig. 2g ) and endonuclease activity ( Fig. 2h ) was substantially reduced by this mutation. Surprisingly, the mutant exhibited similar dsDNA exonuclease activity as that of the wild-type enzyme ( Supplementary Fig. 4 ), suggesting that DNA-induced dimerization endows FAN1 with 5′ flap-structure specific endonuclease activity, while the exonuclease activity may not require dimerization. Interestingly, the mutation R982E on the PVRR NUC side of the interface had no effect on DNA-induced FAN1 dimerization ( Fig. 2f ) and 5′ flap DNA-binding capacity ( Fig. 2g ), but showed a slightly different binding pattern with 5′ flap DNA ( Fig. 2g ). It almost completely ablated both endonuclease and exonuclease activities ( Fig. 2h and Supplementary Fig. 4 ). This indicates that R982E may perturb the dimerization conformation leading to catalytically unproductive DNA binding. FAN1-DNA interface The DNA interaction modules of the FAN1 dimer tether and orient the duplex regions of the 5′ flap DNA substrate ( Fig. 3a–c ) before unwinding and incision. The P SAP surface facing the catalytic site constitutes the major DNA-binding site that recognizes the sugar-phosphate backbone of the duplex region downstream of the 5′ flap (denoted as P Duplex). This surface is the most positively charged and conserved region of FAN1 ( Fig. 3a and Supplementary Fig. 6a ). The binding is achieved through extensive electrostatic attraction and hydrogen bonding interactions ( Fig. 3b ). This P SAP-DNA interaction locates the 5′ flap site at the tip of the P SAP domain ( Figs 1a–c and 3b ). Interestingly, the DNA in the ‘substrate-scanning’ form is in a reversed orientation and consequently directs the 5′ flap away from the VRR_NUC active site ( Fig. 1a ). This suggests that DNA may bind in both orientations but only the correct one can lead to substrate latching and unwinding for subsequent incision. 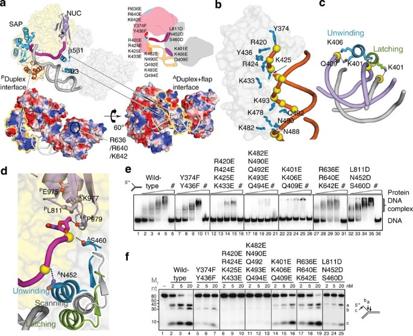Figure 3: The DNA binding modules of FAN1. (a) Overall view of the DNA-binding interface on FAN1 in the ‘substrate-unwinding’ form (top), withPFAN1 as yellow surface andAFAN1 as grey surface. The DNA is shown as grey coils with the flap-containing strand in magenta. The DNA binding modules are highlighted as coloured ribbons withPSAP in cyan (SAP′) and orange (SAP), NUC in violet, and α3and α5β1ofASAP in light cyan and dark cyan, respectively. Bottom: the surface charge distribution of the FAN1 dimer (red: negative; blue: positive). The DNA binding interfaces are marked by yellow borders. The black star marks the active site. The position of the control residues (labelled) used in the mutagenesis study is marked by a black oval. Top right inset: schematic summary of the locations of the mutations included in this figure. (b) Close-up view of thePSAP (grey surface)-PDuplex(orange coils) interaction in the ‘substrate-scanning’ form. DNA-interacting residues are in cyan sticks and phosphate groups are shown as yellow spheres. (c) Close-up view ofASAP-ADuplex interactions (‘substrate-unwinding’ form with protein in cyan, DNA in violet; ‘substrate-latching’ form with protein in green, DNA in grey). The DNA-contacting residues are shown as sticks and phosphates as spheres. (d) Close-up view of the ssDNA-binding interface. The α5β1modules from the ‘substrate-unwinding’ form (cyan), ‘substrate-latching’ form (green) and ‘substrate-scanning’ form (grey) are shown as ribbons. The DNA-binding side chains are shown as sticks (colour scheme: oxygen atoms in red, nitrogen atoms in blue, and carbon atoms from SAP and NUC domains in cyan and light violet, respectively). Transparent surfaces of FAN1 are displayed (PFAN1 in yellow andAFAN1 in grey). (e) DNA mobility shift assay of FAN1373-1,017and its DNA binding mutants using a 5′ flap DNA substrate. (f) Nuclease assay of FAN1373-1,017and its DNA binding mutants. The endo- and exonuclease products were indicated as in (a–c) and shown in the schematic. Quantifications of (e) and (f) are shown inSupplementary Fig. 5. Figure 3: The DNA binding modules of FAN1. ( a ) Overall view of the DNA-binding interface on FAN1 in the ‘substrate-unwinding’ form (top), with P FAN1 as yellow surface and A FAN1 as grey surface. The DNA is shown as grey coils with the flap-containing strand in magenta. The DNA binding modules are highlighted as coloured ribbons with P SAP in cyan (SAP′) and orange (SAP), NUC in violet, and α 3 and α 5 β 1 of A SAP in light cyan and dark cyan, respectively. Bottom: the surface charge distribution of the FAN1 dimer (red: negative; blue: positive). The DNA binding interfaces are marked by yellow borders. The black star marks the active site. The position of the control residues (labelled) used in the mutagenesis study is marked by a black oval. Top right inset: schematic summary of the locations of the mutations included in this figure. ( b ) Close-up view of the P SAP (grey surface)- P Duplex(orange coils) interaction in the ‘substrate-scanning’ form. DNA-interacting residues are in cyan sticks and phosphate groups are shown as yellow spheres. ( c ) Close-up view of A SAP- A Duplex interactions (‘substrate-unwinding’ form with protein in cyan, DNA in violet; ‘substrate-latching’ form with protein in green, DNA in grey). The DNA-contacting residues are shown as sticks and phosphates as spheres. ( d ) Close-up view of the ssDNA-binding interface. The α 5 β 1 modules from the ‘substrate-unwinding’ form (cyan), ‘substrate-latching’ form (green) and ‘substrate-scanning’ form (grey) are shown as ribbons. The DNA-binding side chains are shown as sticks (colour scheme: oxygen atoms in red, nitrogen atoms in blue, and carbon atoms from SAP and NUC domains in cyan and light violet, respectively). Transparent surfaces of FAN1 are displayed ( P FAN1 in yellow and A FAN1 in grey). ( e ) DNA mobility shift assay of FAN1 373-1,017 and its DNA binding mutants using a 5′ flap DNA substrate. ( f ) Nuclease assay of FAN1 373-1,017 and its DNA binding mutants. The endo- and exonuclease products were indicated as in ( a – c ) and shown in the schematic. Quantifications of ( e ) and ( f ) are shown in Supplementary Fig. 5 . Full size image To validate the role of the P Duplex-binding residues on FAN1, we created the following compound mutants: R420E/R424E/K425E/K433E and K482E/N490E/Q492E/K493E/Q494E (the locations of the mutations are shown in Fig. 3a and Supplementary Fig. 2e ). Importantly, both mutants showed significantly impaired binding to 5′ flap DNA and abolished the endonuclease activity ( Fig. 3e,f and Supplementary Figs 4 and 5 ). As a control, a compound mutation, R636E/R640E/K642E, distant from the DNA binding and dimerization interfaces had no effect on DNA-binding capacity or nuclease activity ( Fig. 3a,e,f ). Besides the electrostatic interactions, residues Y374 and Y436 also form two hydrogen bonds with the phosphate backbone of DNA. To validate their functional relevance, we further tested the Y374F/Y436F mutation and the results showed that it retained WT-like 5′ flap DNA-binding affinity but was substantially impaired in endonuclease activity ( Fig. 3e, f ). This indicates that the two residues (Y374 and Y436) may contribute to appropriate substrate orientation through hydrogen-bonding interactions. In addition to the P SAP- P Duplex interaction, A SAP can bind the duplex region upstream of the 5′ flap (denoted as the A Duplex), facilitating the latching and orientation of the DNA ( Fig. 1b,c and Fig. 3c ). This interaction presumably also facilitates DNA-induced FAN1 dimerization. Specifically, A K401 of helix α 3 in A SAP engages the A Duplex in the ‘substrate-latching’ form, and a subsequent ~7 Å translocation of α 3 in the ‘substrate-unwinding’ form generates a tighter contact with the A Duplex through additional contacts involving residues A K409 and A Q406 ( Fig. 3c ). Consistent with the structural observation, the triple mutant K401E/K406E/Q409E of FAN1 showed substantially impaired 5′flap DNA-binding affinity and endonuclease activity ( Fig. 3e and Supplementary Fig. 5 ). The dimerization of FAN1 further creates an interface that facilitates the unwinding of the DNA duplex and guides the liberated ssDNA towards the active site ( Fig. 3d ). The observed ‘unwinding-form’ likely represents a state with partially unwound DNA substrate, as the ssDNA region does not reach the active site for hydrolysis. Further unwinding towards the active site is needed to enable the incision at the previously reported incision point 4 nt downstream of the flap [3] . In the current crystal form, the side chains of A N452 from α 3 and A S460 from α 5 β 1 and the backbone carbonyl of P P979 provide three hydrogen bonds to the backbone of the ssDNA, while P L811 forms stacking interaction with a ribose ring. The compound mutation N452D/S460D/L811D led to substantially impaired nuclease activity ( Fig. 3f ) while preserving near-wild type binding affinity to 5′ flap DNA ( Fig. 3e ). This is consistent with the important role of these residues in guiding the ssDNA region to the active site in P VRR_NUC. The energy needed to unwind the duplex region may be generated by the extra interface of both the A FAN1-DNA interaction and the FAN1 dimerization (additional area of 1,200 Å 2 ) as a result of the change from the ‘latching form’ to the ‘unwinding form’. To further examine the requirement of flap unwinding in incision and to directly assess FAN1’s capacity of ICL unhooking, we designed a series of DNA substrates with a single ICL created by the chemical crosslinker psoralen at various positions relative to the flap. A single ICL at the branch point will prevent the unwinding of the duplex downstream of the 5′ flap, and it also abrogated FAN1 endonuclease cleavage ( Fig. 4a ). To determine how many base pairs must be unwound to allow FAN1 cleavage, the ICL was moved 2, 6, 12 or 16 base pairs away from the flap branch point. Strong inhibition of endonucleolytic incision was observed until the ICL was 6–12 base pairs or further away from the flap site ( Fig. 4b ), which is consistent with the flap unwinding observed in our ‘substrate-unwinding’ structure. 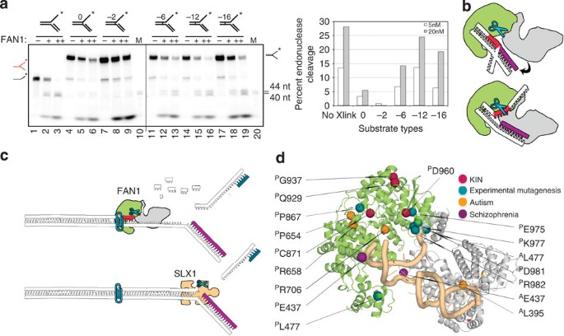Figure 4: FAN1 in ICL repair and related disorders. (a) Nuclease assay of FAN1373-1,017,(at the concentrations of 0 nM labelled as ‘−’, 5 nM as ‘+’, and 20 nM as ‘++’) on 5′ flap DNAs crosslinked at different positions. Endonuclease products are indicated with molecular weight standard (M). The location for the predicted cleavage product of crosslinked DNA (at 0 and −2 positions) is marked by red schematic. Note the absence of the product. Left: gel image; right: quantification of the cleavage product. (b) Schematic for the unwinding-incision action of FAN1 (PFAN1 in light-green,AFAN1 in grey and the active site indicated by cyan scissors). The unwinding region is in red, the antisense strand in the duplex region is in magenta and the rest of DNA is in white. (c) Schematics for the comparison of FAN1 (top) and SLX1 (bottom) in processing DNA lesions at various positions away from the ICL. (d) The structural mapping of the reported deleterious mutants of FAN1 in the ‘substrate-unwinding’ form (PFAN1 in light green,AFAN1 in grey and DNA in light orange. KIN: karyomegalic interstitial nephritis). The Cα of the missense residues are labelled and highlighted as spheres (coloured in a source-specific scheme as indicated). Figure 4: FAN1 in ICL repair and related disorders. ( a ) Nuclease assay of FAN1 373-1,017, (at the concentrations of 0 nM labelled as ‘−’, 5 nM as ‘+’, and 20 nM as ‘++’) on 5′ flap DNAs crosslinked at different positions. Endonuclease products are indicated with molecular weight standard (M). The location for the predicted cleavage product of crosslinked DNA (at 0 and −2 positions) is marked by red schematic. Note the absence of the product. Left: gel image; right: quantification of the cleavage product. ( b ) Schematic for the unwinding-incision action of FAN1 ( P FAN1 in light-green, A FAN1 in grey and the active site indicated by cyan scissors). The unwinding region is in red, the antisense strand in the duplex region is in magenta and the rest of DNA is in white. ( c ) Schematics for the comparison of FAN1 (top) and SLX1 (bottom) in processing DNA lesions at various positions away from the ICL. ( d ) The structural mapping of the reported deleterious mutants of FAN1 in the ‘substrate-unwinding’ form ( P FAN1 in light green, A FAN1 in grey and DNA in light orange. KIN: karyomegalic interstitial nephritis). The Cα of the missense residues are labelled and highlighted as spheres (coloured in a source-specific scheme as indicated). Full size image The current model for ICL repair posits that the replication forks converge onto the ICL, producing an ICL flanked by two DNA flaps (3′ and 5′) that must be unhooked by two incisions, one at the base of each flap [17] , [18] . SLX1, another 5′ flap endonuclease, and FAN1 are thought to play overlapping roles in 5′ flap processing during ICL repair [4] , [18] , [19] . However, while SLX1 cuts the ssDNA flap at the branch point [20] , FAN1 can create incisions both on the ssDNA flap and within the duplex region downstream ( Fig. 2 and Supplementary Fig. 2 ) [3] , [12] . This could be explained by the unwinding of duplex DNA followed by incision of the unwound ssDNA ( Fig. 4a ), as suggested by our structural and biochemical data. FAN1 would mediate DNA incision further away from the ICL ( Fig. 4c ). The involvement of FAN1 and SLX1 in ICL repair would expand the repair spectrum and properly incise various DNA structures or at different steps of ICL repair. SLX1 has been proposed to play a prominent role in ICL unhooking [18] , while FAN1 may be more involved in the homologous recombination reaction during ICL repair [1] , [18] , [21] . The active site and the P Duplex interfaces of FAN1 are evolutionarily conserved from bacteria to humans, while the protein dimerization, DNA flap binding and A Duplex interfaces appear to be unique to higher eukaryotic species ( Supplementary Figs 6 and 7 ). In particular, the core α 9 helix (bearing residues K525, R526 and K528), essential for dimerization and nuclease activity in human FAN1, is substantially shorter or absent in lower species ( Supplementary Figs 6b,c and 7 ). This suggests that bacterial FAN1 orthologues may use a different mechanism for DNA binding without protein dimerization. This difference may be due to the fact that eukaryotic FAN1 has evolved to work with other cellular factors, as it is recruited to ICL sites via the monoubiquitinated FANCI/D2 complex [1] , [2] , [3] , [4] , [5] , [6] . Moreover, the FANCI/D2 complex has been shown to interact with branched DNA mainly on the exposed positively charged surface of the protein complex [22] . Our structures reveal that human FAN1 also engages DNA in a relatively open conformation that would allow access by other binding partners. This lends support to the potential simultaneous and collaborative binding of FAN1 and FANCI/D2 to a stalled replication fork during its repair, as proposed previously [2] , [3] , [4] . The FANCI/D2-dependent ICL repair pathway is absent in bacteria, and different catalytic properties for bacterial and human FAN1 have indeed been reported recently [12] . FAN1 mutations [7] , [8] have been implicated in ageing and developmental disorders including chronic kidney disease [7] and mental ailments [8] . In this regard, FAN1 could help ensure organ health by minimizing the harmful effects of genotoxins to which the kidney is exposed and of potential ICL inducers in embryonic neural tissues during the period of rapid genome replication [23] . The elucidation of the human FAN1-DNA structure allows us to assess the existing disease-associated FAN1 variants [7] , [8] via structural mapping ( Fig. 4d ). Mutations of active site residues (D960 (refs 1 , 2 , 7 ), K977 (refs 2 , 24 ), D981 (ref. 3 ), R982 (ref. 3 ), and E975 (ref. 24 )) are expected to abrogate the nuclease activity, while mutations of residues located in the interior of FAN1 (G937 (ref. 7 ), Q929 (ref. 7 ), P867 (ref. 8 ), P654 (ref. 8 ), R658 (ref. 7 ) and C871 (ref. 7 )) could affect protein folding and thus disrupt the structural integrity of FAN1. Moreover, mutations of residues located on the protein dimerization (L477 (ref. 5 ), E437 (ref. 8 ) and R982 (ref. 3 )) and DNA binding (E437 (ref. 8 ), L395 (ref. 8 ), R706 (ref. 8 ) and L477 (ref. 5 )) interfaces likely perturb the dimer structure and impair the DNA-binding activity of FAN1. FAN1 expression has been found to correlate with treatment outcome in breast and ovarian cancers, with increased FAN1 expression leading to a poorer prognosis [11] . In contrast, suppressed FAN1 recruitment to DNA lesions may account for the enhanced response to ICL-inducing chemotherapy drugs in lung cancer [10] . In these regards, FAN1 is a promising target for improving chemotherapy efficacy. Results from our study establish a structural and biochemical basis for understanding human disorders caused by FAN1 deficiency and for the potential design of new anticancer treatments targeting FAN1. Cloning, expression and purification The full-length human FAN1 gene was cloned into an E. coli expression vector pET43.1. Site-directed mutagenesis on D960A was introduced before subcloning for structural studies. FAN1 373-1,017 D960A was subcloned into the pMAT9s expression vector containing a N-terminal 6xHis tag followed by the maltose binding protein (MBP) and a SARS-CoV M pro cleavage site [25] , [26] . The protein was expressed in the E. coli strain BL21 (DE3) by a 16-h induction with 0.1 mM isopropyl β-D-thiogalactopyranoside (IPTG) at 16 °C and a starting cell density of OD 600 of 0.8. The protein was purified using amylose agarose beads (GE Healthcare) and Superdex 200 size exclusion column. Homogenous fractions of FAN1 protein were collected and concentrated to 5 mg ml −1 in protein storage buffer (20 mM Tris pH 8.0, 1 M NaCl, 50% glycerol) at −80 °C. FAN1 mutants were generated using the QuickChange site-directed mutagenesis kit (Stratagene), verified by DNA sequencing, expressed and purified using the same procedure described above. Notably, all mutants used throughout the study were purified as monodispersed monomers and displayed identical chromatographic behaviour, indicating the overall folding of the protein is not perturbed by any of the mutations. FAN1-DNA complex preparation and purification 5′ Flap DNA substrates were prepared by mixing equimolar amounts of DNA oligonucleotides (a3-10-1/b22(AT)/c10 for the ‘substrate-scanning’ form and a3-10-1/b22/c10 for the ‘substrate-latching’ and ‘substrate-unwinding’ forms; sequences of the oligonucleotides are in Supplementary Table 1 ) were mixed in a buffer containing 20 mM Tris-HCl, pH 8.0, 100 mM NaCl, 5 mM MgCl 2 , 0.1 mM Tris (2-chloroethyl) phosphate (TCEP) at 95 °C, followed by slow annealing from 95 °C to 4 °C over 16 h. The annealed product was purified using a Superdex 200 size exclusion column, concentrated to 0.5 mM and stored at −20 °C. For crystallization, the 6xHis-MBP tag was cleaved from FAN1 373-1,017 D960A by the SARS-CoV M pro protease. FAN1 373-1,017 (D960A)-DNA complex was obtained by mixing protein with DNA substrate at 1:1 molar ratio and purification by gel-filtration chromatography in a Superdex 200 column in 20 mM Tris-HCl, pH 8.0, 50 mM NaCl and 0.1 mM TCEP. Complex fractions were collected, concentrated to 5 mg ml −1 and stored at −80 °C. Crystallization and structure determination The FAN1–DNA complexes were crystallized using the macro-batch under oil method [27] at room temperature. A mixture of protein and reservoir buffer was deposited under a layer of 2:1 paraffin (Fluka):silicon (Hampton Research) oil and allowed to equilibrate at room temperature. Crystals of the ‘substrate-scanning’ form were obtained in a crystallization buffer containing 210 mM potassium iodide, 100 mM Bis-Tris-HCl, pH 7.3, with 18% PEG 3350, and 2 mM spermidine. The crystals were cryo-protected using the crystallization solution containing 25% glycerol and then frozen in liquid nitrogen. Data sets were collected at NE-CAT beamline 24ID-C at the Advanced Photon Source, Argonne National Laboratory, and beamlines X29 and X25 at the National Synchrotron Light Source, Brookhaven National Laboratory. Anomalous signals from the iodine ions were carefully collected using a low-dose shutter-less data collection strategy at the wavelength of 1.595 Å ( f ′′=7.3 for iodine). Five isomorphous data sets from three crystals were processed, merged and scaled in space group P2 1 2 1 2 1 to 2.8 Å resolution using XDS [28] ( Table 1 ), with useful anomalous signal existing to 4 Å, where the Pearson correlation coefficients [29] CC 1/2 =0.99 and CC Anom =0.2 in the resolution shell 4.4–4.0 Å. A total of 11 iodine sites were located using SHELX [30] and initial phases were determined by the SAD method using Phenix [31] and SHARP [32] . Subsequent density modification in SHARP produced an excellent electron density map in which unambiguous protein and DNA features were easily discernable ( Supplementary Fig. 1 ). An initial model of the FAN1 molecule and entire duplex region of the DNA substrate was built using a combination of automated model building by Buccanneer [33] and manual rebuilding in Coot [34] . A slightly non-isomorphous native data set was subsequently collected at 0.9792 Å wavelength to a resolution of 2.2 Å by merging five data sets from three crystals. The structure was solved using the initial FAN1-DNA model by molecular replacement using Phaser [35] and refined to a final R / R free of 0.220/0.256 using Refmac [36] , [37] with good Ramachandran statistics (95.3% favoured, 4.0% allowed, 0.7% outliers). Crystals of the ‘substrate-latching’ and ‘substrate–unwinding’ forms were grown in the same manner as the ‘substrate-scanning’ form, but were in space group P3 1 and diffracted to modest resolutions of 4.2 and 3.8 Å, respectively. A thorough inspection of the diffraction data revealed that both crystals were twinned, with twinning fractions ~0.4 ( Table 1 ). Both the conventional twinning test, such as cumulative intensity distribution, the L test [38] and the maximum likelihood method implemented in Phenix. Xtriage [31] clearly revealed twinning with the twining operator ‘ h,-h-k,-l ’ ( Supplementary Fig. 8 ). Each crystal form contained two FAN1 molecules and one DNA in the asymmetric unit and the structures were solved by molecular replacement in Phenix , using the FAN1 model obtained in the P2 1 2 1 2 1 crystal and ideal B-DNA models. After successful amplitude-based twin refinement in Refmac5 [37] , unbiased difference electron density for the ssDNA region appeared in the ‘substrate-unwinding’ form before the inclusion of the ssDNA model ( Fig. 1e ). Iterative model rebuilding in Coot and refinement in Refmac5 produced the final models of R / R free =24.8/28.3% for the ‘substrate-unwinding’ form (Ramachandran statistics: 94.0% favoured,4.3% allowed, 1.7% outliers) and R / R free =23.5/28.8% for the ‘substrate-latching’ form (Ramachandran statistics: 96.0% favoured, 3.0% allowed, 1.0% outliers). We further calculated simulated-annealing composite-omit difference Fourier maps and the results clearly validated the different DNA conformations observed in the ‘substrate-latching’ and ‘substrate-unwinding’ forms ( Supplementary Fig. 1 ). DNA substrates for biochemical assays All the substrates were made by annealing of a 5′ 32 P-labelled oligonucleotide with the complementary unlabelled oligonucleotide(s) (sequence details in Supplementary Tables 1 and 2 ). The oligonucleotides M34 to M46 (lengths from 34 to 46 nt) were derived from the oligonucleotide H3 and were used as radioactive markers in gel analysis to determine the endonuclease incision sites. The annealed DNA substrates were then purified by electrophoresis on a native 8% polyacrylamide gel and recovered by the crushing and soaking method. Psoralen-crosslinked DNA preparation and purification Oligonucleotides (X0F, X2F, X6F, X12F and X16F, Supplementary Table 1 ) were 32 P-labelled at the 5′ end of the strand constituting the 5′ flap. Labelled oligonucleotides were annealed with the complementary partner (2 μM each, Supplementary Table 2 ) in annealing buffer (10 mM Tris-HCl, pH 8.0, 100 mM NaCl, 1 mM EDTA, 2.5 mM MgCl 2 ) to generate splayed arm structures. A total of 412.5 μM 4′-Hydroxymethyl-4, 5′, 8-trimethylpsoralen (Berry and Associates, Dexter, MI) was added to the annealed oligonucleotides, incubated at room temperature for 1 h, and the mixture was then exposed to UVA light (1.12 J cm −2 ) for 15 min to crosslink the complementary strands at the unique TpA site in each substrate. The DNA preparation was resolved in an 8% denaturing gel, whereupon the crosslinked species was excised, electroeluted and concentrated (Amicon Ultra 10,000 MWCO filtration device). The crosslinked species were then annealed with the third strand (X40, Supplementary Table 1 ) in annealing buffer. In parallel, a substrate without any crosslink was generated by annealing oligonucleotides X0F, X0R and X40. Nuclease assays FAN1 373–1,017 (2, 5, 20 nM or as indicated) with 5 nM of radiolabelled DNA substrates (5′-flap, 3′-flap, dsDNA or dT80) at 37 °C in buffer R (20 mM Tris-HCl, pH 7.5, 5 mM MgCl 2 , 1 mM DTT, 0.05 mg ml −1 BSA, 15 mM KCl) for 5 min. DNA substrates containing a psoralen crosslink were tested with 5 and 20 nM of FAN1 in the same manner. The reactions were stopped by the addition of 10 mM EDTA. Following deproteinization by treatment with SDS (0.5% final) and proteinase K (0.5 mg ml −1 ) for 5 min at 37 °C, the reactions were heated at 95 °C for 5 min and resolved in a denaturing gel (9% polyacrylamide and 8 M urea) in TBE buffer (45 mM Tris-borate, 1 mM EDTA, pH 8.0) at 55 °C. Gels were dried onto Whatman DE81 paper (Whatman International Limited) and analysed in a Personal Molecular Imager FX PhosphorImager (Bio-Rad). Quantification data were expressed as average with s.d. values from triplicated experiments. BMH protein crosslinking assay FAN1 373-1,017 or its mutant (1.37 μM) was pre-incubated with or without a 5′ flap DNA (10-1-10) substrate (0.27 and 1.37 μM) at room temperature for 10 min in 10 μl of buffer (20 mM Hepes, pH 7.2, 5 mM EDTA, 5 mM MgCl 2 , 95 mM KCl). The crosslinking reaction was conducted by the addition of 4 μM BMH (bis(maleimido)hexane, Pierce) at 25 °C for 10 min and was stopped by the addition of 15 mM DTT. The reaction mixtures were then resolved in 4–15% SDS–polyacrylamide gel electrophoresis (SDS–PAGE) and silver stained. DNA mobility shift assay FAN1 373-1,017 wild type or mutant (20, 40, 80 and 120 nM) was incubated with the radiolabelled 5′-flap DNA substrate (5 nM) at 37 °C for 10 min in 10 μl of buffer D (30 mM Tris-HCl, pH 7.5, 1 mM DTT, 100 μg ml −1 BSA and 15 mM KCl). The reaction mixtures were resolved in 6.5% polyacrylamide gels at 4 °C in TBE buffer. Gels were dried and analysed in the PhosphorImager. Quantification data were expressed as average with stand deviations from triplicated experiments. SEC-MALLS (Multi-angle laser light scattering) assay SEC-MALLS data were collected using an Ettan LC system (GE Healthcare) with a Superdex 200 Increase 10/300 column (GE Healthcare) equilibrated in buffer E (20 mM Tris HCL, pH 8.0, 80 mM NaCl, and 0.1 mM TCEP) at a flow rate of 0.5 ml min −1 . The system was coupled on-line to an 18-angle MALLS detector and a differential refractometer (DAWN HELEOS II and Optilab rEX, Wyatt Technology). Molar mass determination was calculated with ASTRA 6.2 software. How to cite this article: Zhao, Q. et al . Structural insights into 5′ flap DNA unwinding and incision by the human FAN1 dimer. Nat. Commun. 5:5726 doi: 10.1038/ncomms6726 (2014). Accession codes: The atomic coordinates and structure factors for the three FAN1-DNA crystal forms have been deposited in the Protein Data Bank with accession codes: 4REA (unwinding form), 4REB (latching form), 4REC (scanning form).